Kinetically tuned dimensional augmentation as a versatile synthetic route towards robust metal–organic frameworks Metal–organic frameworks with high stability have been pursued for many years due to the sustainability requirement for practical applications. However, researchers have had great difficulty synthesizing chemically ultra-stable, highly porous metal–organic frameworks in the form of crystalline solids, especially as single crystals. Here we present a kinetically tuned dimensional augmentation synthetic route for the preparation of highly crystalline and extremely robust metal–organic frameworks with a preserved metal cluster core. Through this versatile synthetic route, we obtain large single crystals of 34 different iron-containing metal–organic frameworks. Among them, PCN-250(Fe 2 Co) exhibits high volumetric uptake of hydrogen and methane, and is also stable in water and aqueous solutions with a wide range of pH values. Metal–organic frameworks (MOFs) with good stability have been pursued for many years [1] , [2] , [3] , [4] . Chemically stable MOFs, which are resistant to reactive species, are of critical importance to a variety of applications, including gas storage, carbon capture, separations and catalysis [5] , [6] , [7] , [8] , [9] , [10] , [11] , [12] , [13] , [14] , [15] . In particular, robust MOFs that are easy to scale up and moisture-resistant with high gas storage capacity are needed for automotive applications. However, making robust MOFs with desired structure, porosity and internal surface properties has always been a challenge. Almost all MOFs, in particular moisture-resistant MOFs constructed with high-valence metal ions, have been made from the ‘one-pot’ synthetic route, making it difficult to control the metal-containing nodes and therefore the topology of the MOF [16] . Problems arise when targeting chemically stable MOFs through conventional one-pot reactions: The overall design of novel MOFs with expected structures, even simple functionalization of existing MOFs for targeted applications, becomes very challenging because of the unpredictable in situ formation of inorganic building blocks; mixed phases often come out together due to the formation of diverse inorganic building blocks; polycrystalline or even amorphous products are prone to form [17] , which not only bring challenges in structure determination, but also influence the properties of the targeted products. To address these problems, we present a general method, which is derived from the rationalization of the MOF growth process from both a kinetic and a thermodynamic perspective, of synthesizing Fe-MOF single crystals with preformed inorganic building blocks [Fe 2 M(μ 3 -O)(CH 3 COO) 6 ] (M=Fe 2+,3+ , Co 2+ , Ni 2+ , Mn 2+ , Zn 2+ ). Overall, we synthesize large single crystals of 34 different Fe-MOFs with thirty different ligands and mixed ligands by rationally tuning the synthetic conditions. Among them, PCN-250(Fe 2 Co) (PCN stands for porous coordination network), which is stable in H 2 O for more than 6 months, exhibits not only one of the highest total CH 4 uptakes of 200 V STP/V at 35 bar and 298 K, but also one of the highest total H 2 volumetric uptakes of 60 g L −1 at 40 bar and 77 K (refs 18 , 19 ). Rationalization of kinetics in the MOF growth process Most chemically stable MOFs are constructed with hard Lewis acidic metal ions such as Fe 3+ , Al 3+ and Zr 4+ when carboxylate ligands (hard bases) are used [20] , [21] , [22] , [23] , [24] , [25] . Due to the strong electrostatic interaction between the metal nodes and organic linkers, the frameworks are relatively resistant to the attack of H 2 O and acidic or basic reactants. However, the stronger coordination bond is also more difficult to dissociate during the MOF growth process, which results in insufficient structure reorganization or defect reparation. As a result, highly crystalline stable MOFs are extremely difficult to synthesize under normal conditions. The MOF crystal growth process is essentially ligand substitution on metal ions or clusters. As most substitution reactions of octahedral complexes go through a dissociative mechanism, ligand substitution reactions (X: initial coordinating ligand, L: bridging ligand) on each individual inorganic building block during MOF growth can be modelled as the stepwise substitution on metal or metal clusters (M; Supplementary Fig. 1 ) The model in Supplementary Fig. 1 illustrates how we can tune the synthesis conditions to promote the flux of ligands on and off a metal cluster and hence facilitate defect reparation and structure reorganization. Consider a metal cluster fully bound to only initial coordinating ligands. The rate of substitution for one of the initial coordinating ligands with a bridging ligand ( r s1 ) At steady state, Thus, X behaves as a competitor to L, and we can slow the rate of bridging ligand attachment by increasing the concentration of X . For the dissociation process of the bridging ligand, the reaction rate is For relatively soft Lewis acidic species such as Cu 2+ and Zn 2+ , interactions with hard basic carboxylates are relatively weak, so the activation energy E a for the dissociation process is small, which yields a large k −2 and a fast dissociation process. Meanwhile, the excess of solvent molecules could serve as an X ligand to compete with the bridging ligand L , which slows down the ligand substitution process. Consequently, ligand substitution and dissociation rates are comparable, allowing sufficient structure reorganization and defect reparation to form long-range ordered structures under moderate conditions. For hard Lewis acidic species such as Fe 3+ , Al 3+ and Zr 4+ , their strong electrostatic interaction with the hard basic carboxylate gives rise to a much larger E a and smaller k −2 . Even if solvent molecules act as an X ligand, the much larger k 1 value still causes unbalanced substitution and dissociation reaction rates. As a result, direct synthesis of those MOFs usually results in a long-range disordered (amorphous) product due to the lack of structural reorganization. Since E a is determined by the nature of the metal and the coordinating ligand, increasing the synthetic temperature T is an approach to raise k −2 and facilitate the ligand dissociation process. Unfortunately, higher temperatures also accelerate the substitution process and an unbalanced substitution–dissociation process still exists. To accelerate the ligand dissociation process at higher temperature and maintain a slow ligand substitution process, an extra competing reagent X , which binds more strongly to the metal (smaller k 1 ) than the solvent molecule is necessary. With the assistance from the extra competing reagent X , reversible ligand rearrangement could be tuned to facilitate the crystallization process [26] , [27] . Because it is actually the carboxylate and not the acid doing the substitution, when the deprotonation process is taken into account, extra acetic acid could simultaneously inhibit the deprotonation of the ligand, which further slows down the substitution reaction and aids the crystallization process. Simplification of MOFs growth using preformed [Fe 2 M(μ 3 -O)( CH 3 COO) 6 ] As M 3 (μ 3 -O)(COO) 6 (M=Fe, Cr, Al, Sc, V, In) is one of the most common building blocks in the reported trivalent metal species containing MOFs [28] , to test our hypothesis, we used [Fe 2 M(μ 3 -O)( CH 3 COO) 6 ] as the starting material and acetic acid (acetate after deprotonation) as the competing reagent to grow Fe-MOFs with many different ligands ( Supplementary Methods ). [Fe 2 M(μ 3 -O)(CH 3 COO) 6 ] as isolated basic carboxylates have been reported for decades [29] . Excellent solubility of these clusters increases their feasibility as a starting material. Meanwhile, due to the strong electrostatic interaction between Fe 3+ and μ 3 -O 2− , the cluster is inherently robust enough to preserve the integrity of the core while going through carboxylate substitution on the periphery under solvothermal conditions. Moreover, the D 3h cluster itself possesses six carboxylate arms in a trigonal prismatic arrangement, which allows facile construction of three-dimensional frameworks through simple bridging. When [Fe 2 M(μ 3 -O)(CH 3 COO) 6 ] is used as a starting material, direct synthesis of Fe-MOFs can be considered as a pure ligand substitution process and the framework growth can be rationalized by a traditional stepwise ligand substitution reaction model ( Supplementary Methods ). Therefore, the addition of extra competing reagent can tune both ligand substitution and dissociation processes directly via concentration variation. Consequently, with the assistance of acetic acid as a competing reagent, we obtained large single crystals of 34 Fe-MOFs containing the [Fe 2 M(μ 3 -O)] building block ( Supplementary Data 1 , Supplementary Figs 2–36 , Supplementary Tables 1–31 , Supplementary Note 1 ). Even though the ligands shown in Fig. 1b vary in symmetry, functionality, connectivity and size, the structure of the [Fe 2 M(μ 3 -O)] building block is maintained in these frameworks. Thus, the new synthetic strategy can be viewed as a dimensional augmentation process from zero-dimensional metal-containing nodes of [Fe 2 M(μ 3 -O)] to three-dimensional nets. Partial substitution on the [Fe 2 M(μ 3 -O)] clusters has also occurred when complete substitution becomes incompatible with some of the ligands because of symmetry requirements or steric hindrance. 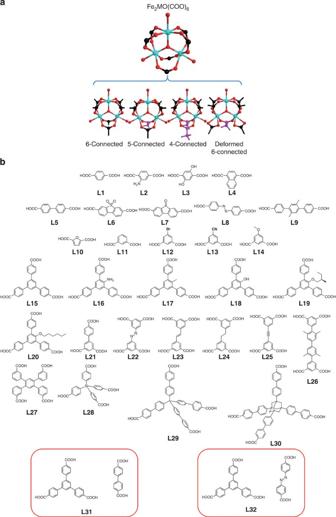Figure 1: Organic linkers used and different connecting modes. (a) Four different connecting modes of the [Fe2M(μ3-O)] cluster. Carboxylates on ligands and terminal acetates are represented by black and purple, respectively. (b) Thirty different ligands and two types of mixed ligands used in constructing Fe-MOFs. Figure 1: Organic linkers used and different connecting modes. ( a ) Four different connecting modes of the [Fe 2 M(μ 3 -O)] cluster. Carboxylates on ligands and terminal acetates are represented by black and purple, respectively. ( b ) Thirty different ligands and two types of mixed ligands used in constructing Fe-MOFs. Full size image To demonstrate our versatility of the kinetically tuned dimensional augmentation strategy, MOFs with distinct structural features are discussed in detail. PCN-240, constructed from L3 , is isostructural to MIL-88 with the acs-a topology ( Fig. 2a ) [3] . Usually, L3 tends to form the MOF-74 structure with two hydroxyl groups participating in coordination. However, when starting from [Fe 2 M(μ 3 -O)(COOCH 3 ) 6 ], the in situ formation of the one-dimensional chain can be avoided and only a simple substitution reaction occurs between carboxylates, leaving two hydroxyl groups free for other potential modifications. With elongated ligands L5 and L9 , which allows sufficient space for catenation, twofold perpendicular interpenetration and threefold parallel interpenetration have been observed, respectively. Interestingly, the interpenetration restricts the flexibility in each single net and therefore stabilizes the framework and generates permanent porosity ( Fig. 2a ). The mixed ligand strategy is challenging due to the high probability of obtaining mixed phases, especially for MOFs on the basif of high-valence metals whose structure determination relied almost exclusively on powder X-ray diffraction. When starting with pre-assembled metal clusters, the interference from side reactions generating different inorganic building blocks is eliminated. The mixed ligand MOFs can be more easily synthesized with the kinetically tuned dimensional augmentation strategy, which allows for growing single crystals instead of powders. Using the combinations of L15 and L5 , as well as L15 and L8 , we obtained large single crystals of PCN-280 and PCN-285 ( Fig. 2b ). 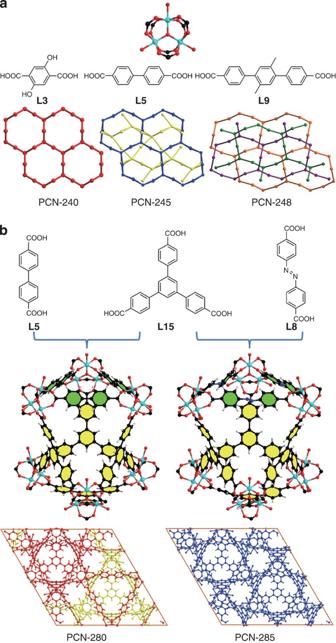Figure 2: Functionalization and mixed ligands in Fe-MOFs. (a) Functionalized MIL-88 isostructure, 2-fold and 3-fold self-interpenetration. (b) PCN-280(interpenetrated) and PCN-285(non-interpenetrated) constructed from mixed ligands. Figure 2: Functionalization and mixed ligands in Fe-MOFs. ( a ) Functionalized MIL-88 isostructure, 2-fold and 3-fold self-interpenetration. ( b ) PCN-280(interpenetrated) and PCN-285(non-interpenetrated) constructed from mixed ligands. Full size image PCN-234 is isostructural to MIL-59 with the CaB 6 net ( Fig. 3a ) [30] . When the ligand is functionalized by bulky groups like -CN, the limited distance between each ligand prevents complete substitution on the [Fe 2 M(μ 3 -O)] cluster and forces the formation of a 5-connected cluster with acetic acid as the remaining terminal ligand ( Fig. 3b ), giving rise to PCN-236. This connectivity reduction also occurs with the tetrahedral ligands: in PCN-265, L29 slightly stretches from the ideal T d symmetry to D 2d symmetry to form a 6-connected [Fe 2 M(μ 3 -O)]-containing framework, while the smaller tetrahedral ligand L28 is too rigid to bend and maintains the original T d symmetry in PCN-264. Complete substitution on the [Fe 2 M(μ 3 -O)] core is unable to form a long-range ordered structure with T d symmetric L28 , so the connectivity of the [Fe 2 M(μ 3 -O)] cluster is reduced to four ( Fig. 3c ). This reduced connectivity on the [Fe 2 M(μ 3 -O)] cluster is first discovered here in these Fe-MOFs, which is also an evidence of the substitution reaction of the preformed basic carboxylate. 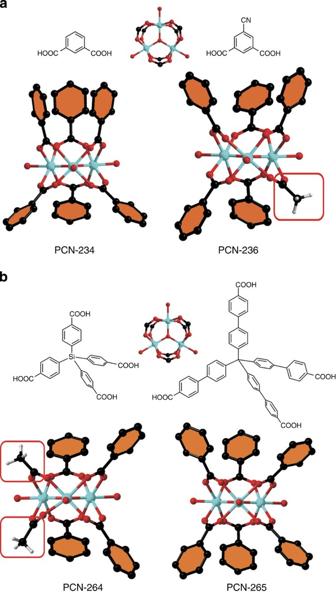Figure 3: Partially substituted [Fe2M(μ3-O)] in Fe-MOFs. (a) Bulky group induced partial substitution in PCN-236. (b) Rigidity induced partial substitution in PCN-264. Figure 3: Partially substituted [Fe 2 M(μ 3 -O)] in Fe-MOFs. ( a ) Bulky group induced partial substitution in PCN-236. ( b ) Rigidity induced partial substitution in PCN-264. Full size image Although all the Fe-MOFs are synthesized under similar conditions, the optimal concentration of acetic acid for each one varies greatly. According to our rationalization, extra acetic acid should slow down the substitution reaction rate, which shows the kinetic influence. When the concentration of acetic acid was much lower than the optimal value, gels or amorphous products were obtained, which suggests insufficient control of the substitution and dissociation balance ( Supplementary Methods ). When the concentration of acetic acid is too high, solutions remain clear with no solid products even after a long period, which suggests a thermodynamic equilibrium in the solution. If MOF formation is expressed as an equilibrium ( Supplementary Fig. 37 ) and the formation of clear solution is treated as the point of a positive Gibbs free energy, then the amount of acetic acid is actually an indication of relative values for the framework’s free energy of formation. The entropic effects can be clearly observed from the synthetic conditions ( Supplementary Table 32 ). For ligands with similar size and connectivity, MOFs containing Fe 2 MO clusters with lower connectivity always need a lower concentration of acetic acid as the competing reagent. Meanwhile, for Fe 2 MO clusters with the same connectivity, ligands with higher connecting numbers always need more acetic acid. Assuming these MOFs have similar enthalpies of formation, the concentration change of acetic acid is consistent with the entropy change. Moreover, even if the connectivity of clusters and ligands are the same, the amount of acetic acid for those MOFs still varies ( Supplementary Table 33 ), which could be attributed to an enthalpic effect ( Supplementary Methods ). Methane uptake is highly related to the structure of the porous material used [19] . Because of the structural diversity of the Fe-MOFs synthesized by us, we turned to computational methods to quickly predict their methane uptake ( Supplementary Methods , Supplementary Figs 44–47 ). In addition, we utilize an in silico approach to predict a set of new structures and their methane uptake ( Supplementary Data 2 and Supplementary Methods ). 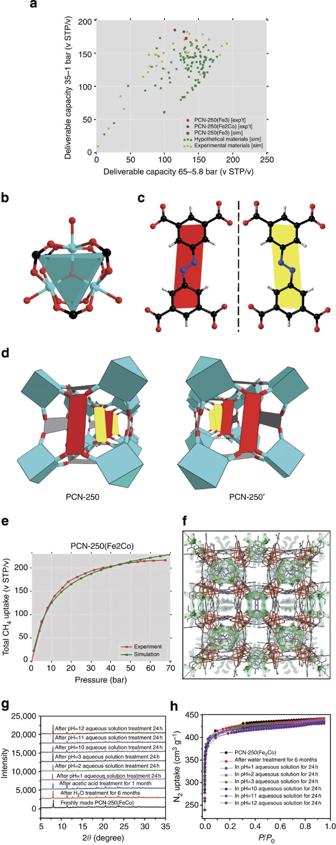Figure 4: Simulated and experimental CH4adsorption of Fe-MOFs. (a) Performance plot of deliverable capacities using two different pressure swings. Shown are the predictions for the Fe-MOFs synthesized here (yellow) andin silicopredicted structures (green). Red and blue points show PCN-250. Our predicted crystal structures and molecular simulation results can be found in theSupplementary Data 1and2. (b–d) Structures of PCN-250 and PCN-250′. (e) Total CH4adsorption uptake of PCN-250 at 298 K and (f) contours of the computed potential energy surface of adsorbed CH4in PCN-250. (g) Powder X-ray patterns and (h) N2adsorption isotherms of PCN-250(Fe2Co) after stability tests. Figure 4a shows the simulated deliverable capacities of our predicted structures and those structures that have been synthesized together with the experimental data of PCN-250(Fe 3 ) and PCN-250(Fe 2 Co). Our simulations suggest that PCN-250 is indeed an outlying structure for vehicular methane storage using a 35–1 bar pressure swing. Interestingly, our screening predicts that several of the synthesized Fe-MOFs have very high deliverable capacities using a 65–5.8 bar pressure swing. Also, our simulations confirm that PCN-250 has the highest 35 bar loading of all structures considered in this analysis ( Supplementary Figs 42 and 43 ). Figure 4: Simulated and experimental CH 4 adsorption of Fe-MOFs. ( a ) Performance plot of deliverable capacities using two different pressure swings. Shown are the predictions for the Fe-MOFs synthesized here (yellow) and in silico predicted structures (green). Red and blue points show PCN-250. Our predicted crystal structures and molecular simulation results can be found in the Supplementary Data 1 and 2 . ( b – d ) Structures of PCN-250 and PCN-250′. ( e ) Total CH 4 adsorption uptake of PCN-250 at 298 K and ( f ) contours of the computed potential energy surface of adsorbed CH 4 in PCN-250. ( g ) Powder X-ray patterns and ( h ) N 2 adsorption isotherms of PCN-250(Fe 2 Co) after stability tests. Full size image PCN-250 consists of 6-connected [Fe 2 M(μ 3 -O)] building blocks and rectangular tetratopic L22 ( Fig. 4b–d ), which is isostructural to the reported indium MOF [31] . Interestingly, PCN-250′, another framework isomer of PCN-250, is found under different synthetic conditions ( Supplementary Methods ). Along one axis, ligands constructing the same cube in PCN-250 adopt mirror configurations and are alternatively arranged. In PCN-250′, ligands adopt the same configuration in the one cube and mirror configuration in the adjacent cubes along any axis. Experimental results show PCN-250(Fe 2 Co) that possesses total CH 4 uptake of 200 v/v at 35 bar and 298 K ( Fig. 4e ), which is one of the highest among all the reported MOFs. PCN-250(Fe 2 Co) has a record high H 2 uptake of 3.07 wt% and 28 g L −1 at 1.2 bar and 77 K ( Supplementary Fig. 38 ). It also has one of the highest total volumetric H 2 uptakes, 60 g L −1 ( Supplementary Fig. 41 ), at high pressure due to its high crystal density. Both high uptake of H 2 and CH 4 can be attributed to suitable size of the cage in PCN-250 and the well-dispersed, highly charged open metal sites ( Fig. 4f ). Each cube in PCN-250 is faced by L22 and the channels between each cube are surrounded by high valent open metal sites. Therefore, all of the void space is provided with adsorption sites, which can strongly interact with both H 2 and CH 4 molecules. This results in efficient space utilization to reach a high volumetric uptake and leads to an induced polarization of gas molecules by high-valence metal cations through charge-induced dipole interaction. This high-valence metal ion and induced dipole interaction can polarize additional layers of gas molecules, allowing multiple layers of gas to adsorb without significant drop in the adsorption enthalpy. The heat of adsorption is relatively low compared with a single-site adsorption by orbital interaction, such as the Kubas binding of hydrogen molecules. However, it is far-reaching, making it nearly flat over a wide range of uptakes ( Supplementary Figs 39 and 40 , Supplementary Methods ). Even after the insertion of the softer Lewis acid M(II) in the μ 3 -oxo trimmer, the PCN-250 series still shows extraordinary chemical stability. The powder patterns of PCN-250(Fe 2 Co) remained unaltered upon immersion in glacial acetic acid and pH=1 to pH=11 aqueous solutions for 24 h ( Fig. 4g,h ). The framework of PCN-250(Fe 2 Co) remained stable under H 2 O after 6 months ( Fig. 4g,h , Supplementary Tables 34 and 35 ). Moreover, the N 2 adsorption isotherms of PCN-250(Fe 2 Co) remain constant after all these treatments, which suggest no phase transition or framework decomposition during all the treatments. A combination of high uptake and chemical stability is quite rare for MOFs, and this combination can guarantee the reusability of the sorbent for industrial applications. With its high gas uptake, extraordinary stability and excellent scalability, PCN-250 is a viable candidate for natural gas storage for automotive applications. Preparation of preformed clusters Fe 2 M(μ 3 -O) (CH 3 COO) 6 (abbreviated to Fe 2 M in MOFs’ syntheses) (M=Mn, Co, Ni, Zn) is prepared according to reported procedure [25] : A solution of sodium acetate trihydrate (42 g, 0.31 mol) in water (70 ml) was added to a filtered, stirred solution of iron(III) nitrate nonahydrate (8 g, 0.02 mol) and the metal(II) nitrate (0.1 mol) in water 70 ml, and the brown precipitate was filtered off, washed with water and with ethanol and dried in air. For M=Zn, the total volume of water used in the preparation was restricted to 70 ml and a red-brown precipitate appeared overnight. Synthesis of PCN-233 L10 (15 mg), Fe 2 Co (15 mg) and acetic acid (0.4 ml) in 2 ml of N , N -dimethyl formamide (DMF) were ultrasonically dissolved in a Pyrex vial. The mixture was heated in an oven at 120 °C for 12 h. After cooling down to room temperature, dark brown crystals were collected by filtration. Synthesis of PCN-234 L11 (8 mg), Fe 3 (15 mg) and acetic acid (0.4 ml) in 2 ml of H 2 O were ultrasonically dissolved in a Pyrex vial. The mixture was heated in an oven at 120 °C for 12 h. After cooling down to room temperature, dark brown crystals were collected by filtration. Synthesis of PCN-235 L11 (15 mg), Fe 2 Co (15 mg) and acetic acid (0.2 ml) in 2 ml of DMF were ultrasonically dissolved in a Pyrex vial. The mixture was heated in an oven at 150 °C for 24 h. After cooling down to room temperature, dark brown crystals were collected by filtration. Synthesis of PCN-236 L13 (15 mg), Fe 2 Co (15 mg) and acetic acid (0.1 ml) in 2 ml of DMF were ultrasonically dissolved in a Pyrex vial. The mixture was heated in an oven at 150 °C for 12 h. After cooling down to room temperature, dark brown crystals were collected by filtration. Synthesis of PCN-237 L12 (15 mg), Fe 2 Co (15 mg) and acetic acid (0.2 ml) in 2 ml of N -methyl pyrrolidone (NMP) were ultrasonically dissolved in a Pyrex vial. The mixture was heated in an oven at 150 °C for 12 h. After cooling down to room temperature, dark brown crystals were collected by filtration. Synthesis of PCN-238 L14 (15 mg), Fe 2 Co (15 mg) and acetic acid (0.1 ml) in 2 ml of NMP were ultrasonically dissolved in a Pyrex vial. The mixture was heated in an oven at 150 °C for 12 h. After cooling down to room temperature, dark brown crystals were collected by filtration. Synthesis of PCN-240 L3 (10 mg), Fe 2 Co (10 mg) and acetic acid (0.25 ml) in 2 ml of N , N -diethylformamide and H 2 O (v/v=1/1) were ultrasonically dissolved in a Pyrex vial. The mixture was heated in an oven at 150 °C for 24 h. After cooling down to room temperature, dark brown crystals were collected by filtration. Synthesis of PCN-241 L4 (10 mg), Fe 2 Co (15 mg) and acetic acid (0.8 ml) in 2 ml of DMF were ultrasonically dissolved in a Pyrex vial. The mixture was heated in an oven at 150 °C for 12 h. After cooling down to room temperature, dark brown crystals were collected by filtration. Synthesis of PCN-242 L2 (10 mg), Fe 3 (10 mg) and acetic acid (0.45 ml) in 2 ml of DMF were ultrasonically dissolved in a Pyrex vial. The mixture was heated in an oven at 150 °C for 12 h. After cooling down to room temperature, dark brown crystals were collected by filtration. Synthesis of PCN-243 L8 (10 mg), Fe 3 (10 mg) and acetic acid (0.45 ml) in 2 ml of DMF were ultrasonically dissolved in a Pyrex vial. The mixture was heated in an oven at 150 °C for 48 h. After cooling down to room temperature, dark brown crystals were collected by filtration. Synthesis of PCN-245 L5 (10 mg), Fe 3 (10 mg) and acetic acid (0.15 ml) in 2 ml of DMF were ultrasonically dissolved in a Pyrex vial. The mixture was heated in an oven at 150 °C for 12 h. After cooling down to room temperature, dark brown crystals were collected by filtration. Synthesis of PCN-246 L7 (10 mg), Fe 3 (15 mg) and acetic acid (0.2 ml) in 2 ml of DMF were ultrasonically dissolved in a Pyrex vial. The mixture was heated in an oven at 120 °C for 12 h. After cooling down to room temperature, dark brown crystals were collected by filtration. Synthesis of PCN-247 L6 (10 mg), Fe 3 (15 mg) and acetic acid (0.35 ml) in 2 ml of DMF were ultrasonically dissolved in a Pyrex vial. The mixture was heated in an oven at 150 °C for 12 h. After cooling down to room temperature, dark brown crystals were collected by filtration. Synthesis of PCN-248 L9 (10 mg), Fe 2 Co or Fe 3 (10 mg) and acetic acid (0.25 ml) in 2 ml of NMP were ultrasonically dissolved in a Pyrex vial. The mixture was heated in an oven at 150 °C for 24 h. After cooling down to room temperature, dark brown crystals were collected by filtration. Synthesis of PCN-250 L22 (10 mg), Fe 2 M (Mn, Fe, Co, Ni, Zn) (15 mg) and acetic acid (1 ml) in 2 ml of DMF were ultrasonically dissolved in a Pyrex vial. The mixture was heated in an oven at 140 °C for 12 h. After cooling down to room temperature, dark brown crystals were collected by filtration. Large scale synthesis of PCN-250 L22 (1 g), Fe 2 M (Mn, Fe, Co, Ni, Zn,) (1 g) and acetic acid (100 ml) in 200 ml of DMF were ultrasonically dissolved in a 500 ml Pyrex bottle. The mixture was heated in an oven at 140 °C for 12 h. After cooling down to room temperature, dark brown crystals were collected by filtration. Synthesis of PCN-250′ L22 (10 mg), Fe 2 M (Mn, Fe, Co, Ni, Zn) (15 mg) and acetic acid (1 ml) in 2 ml of NMP were ultrasonically dissolved in a Pyrex vial. The mixture was heated in an oven at 140 °C for 12 h. After cooling down to room temperature, dark brown crystals were collected by filtration. Synthesis of PCN-251 L22 (10 mg), Fe 2 M (Mn, Fe, Co, Ni, Zn) (15 mg) and acetic acid (1 ml) in 2 ml of NMP were ultrasonically dissolved in a Pyrex vial. The mixture was heated in an oven at 140 °C for 12 h. After cooling down to room temperature, dark brown crystals were obtained. Synthesis of PCN252 L23 (10 mg), Fe 2 M (Mn, Fe, Co, Ni, Zn) (10 mg) and acetic acid (0.8 ml) in 2 ml of NMP were ultrasonically dissolved in a Pyrex vial. The mixture was heated in an oven at 150 °C for 12 h. After cooling down to room temperature, dark brown crystals were colllected by filtration. Synthesis of PCN-253 L24 (10 mg), Fe2M (Mn, Fe, Co, Ni, Zn,) (15 mg) and acetic acid (1 ml) in 2 ml of NMP were ultrasonically dissolved in a Pyrex vial. The mixture was heated in an oven at 150 °C for 12 h. After cooling down to room temperature, dark brown crystals were collected by filtration. Synthesis of PCN-254 L25 (10 mg), Fe 2 M (Mn, Fe, Co, Ni, Zn) (15 mg) and acetic acid (1 ml) in 2 ml of NMP were ultrasonically dissolved in a Pyrex vial. The mixture was heated in an oven at 150 °C for 12 h. After cooling down to room temperature, dark brown crystals were collected by filtration. Synthesis of PCN-255 L26 (10 mg), Fe 2 Co (15 mg) and acetic acid (0.5 ml) in 2 ml of NMP were ultrasonically dissolved in a Pyrex vial. The mixture was heated in an oven at 150 °C for 12 h. After cooling down to room temperature, dark brown crystals were collected by filtration. Synthesis of PCN-256 L27 (10 mg), Fe 2 Co (15 mg) and acetic acid (0.4 ml) in 2 ml of NMP and 0.1 ml n-pentanol were ultrasonically dissolved in a Pyrex vial. The mixture was heated in an oven at 150 °C for 12 h. After cooling down to room temperature, dark brown crystals were collected by filtration. Synthesis of PCN-257 L21 (10 mg), Fe 3 (15 mg) and acetic acid (0.4 ml) in 2 ml of NMP and 0.1 ml n-pentanol were ultrasonically dissolved in a Pyrex vial. The mixture was heated in an oven at 150 °C for 12 h. After cooling down to room temperature, dark brown crystals were collected by filtration. Synthesis of PCN-260 L15 (15 mg), Fe 2 Co (5 mg) and acetic acid (0.25 ml) in 2 ml of NMP were ultrasonically dissolved in a Pyrex vial. The mixture was heated in an oven at 150 °C for 24 h. After cooling down to room temperature, dark brown crystals were collected by filtration. Synthesis of PCN-261-NH 2 L16 (15 mg), Fe 2 Co (15 mg) and acetic acid (0.22 ml) in 2 ml of DMF were ultrasonically dissolved in a Pyrex vial. The mixture was heated in an oven at 150 °C for 12 h. After cooling down to room temperature, dark brown crystals were collected by filtration. Synthesis of PCN-261-CH 3 L17 (15 mg), Fe 2 Co (15 mg) and acetic acid (0.2 ml) in 2 ml of DMF were ultrasonically dissolved in a Pyrex vial. The mixture was heated in an oven at 150 °C for 12 h. After cooling down to room temperature, dark brown crystals were collected by filtration. Synthesis of PCN-261-Chiral L19 (15 mg), Fe 2 Co (15 mg) and acetic acid (0.2 ml) in 2 ml of DMF were ultrasonically dissolved in a Pyrex vial. The mixture was heated in an oven at 150 °C for 12 h. After cooling down to room temperature, dark brown crystals were collected by filtration. Synthesis of PCN-262 L18 (10 mg), Fe 2 Ni (10 mg) and acetic acid (0.25 ml) in 2 ml of DMF were ultrasonically dissolved in a Pyrex vial. The mixture was heated in an oven at 150 °C for 12 h. After cooling down to room temperature, dark brown crystals were collected by filtration. Synthesis of PCN-263 L20 (10 mg), Fe 2 Ni (10 mg) and acetic acid (0.3 ml) in 2 ml of DMF were ultrasonically dissolved in a Pyrex vial. The mixture was heated in an oven at 150 °C for 73 h. After cooling down to room temperature, dark brown crystals were collected by filtration. Synthesis of PCN-264 L28 (10 mg), Fe 3 (10 mg) and acetic acid (0.6 ml) in 2 ml of DMF were ultrasonically dissolved in a Pyrex vial. The mixture was heated in an oven at 150 °C for 24 h. After cooling down to room temperature, dark brown crystals were collected by filtration (Yield 80%). Synthesis of PCN-265 L29 (10 mg), Fe 2 Ni (15 mg) and acetic acid (0.43 ml) in 2 ml of DMF were ultrasonically dissolved in a Pyrex vial. The mixture was heated in an oven at 150 °C for 12 h. After cooling down to room temperature, dark brown crystals were collected by filtration. Synthesis of PCN-266 L30 (10 mg), Fe 3 (15 mg) and acetic acid (0.3 ml) in 2 ml of DMF were ultrasonically dissolved in a Pyrex vial. The mixture was heated in an oven at 150 °C for 12 h. After cooling down to room temperature, dark brown crystals were collected by filtration. Synthesis of PCN-280 L5 (10 mg), L15 (10 mg), Fe 3 (10 mg) and acetic acid (0.2 ml) in 2 ml of NMP and 0.1 ml n-pentanol were ultrasonically dissolved in a Pyrex vial. The mixture was heated in an oven at 150 °C for 12 h. After cooling down to room temperature, dark brown crystals were collected by filtration. Synthesis of PCN-285 L8 (10 mg) and L15 (10 mg), Fe 3 (10 mg) and acetic acid (0.2 ml) in 2 ml of NMP and 0.1 ml n-pentanol were ultrasonically dissolved in a Pyrex vial. The mixture was heated in an oven at 150 °C for 12 h. After cooling down to room temperature, dark brown crystals were collected by filtration. MIL-88 synthesis BDC (10 mg), Fe 2 Co or Fe 3 (10 mg) NMP 2 ml and acetic acid (0.2 ml) were ultrasonically dissolved in a Pyrex vial. The mixture was heated in an oven at 150 °C for 12 h. After cooling down to room temperature, dark brown crystals were collected by filtration. How to cite this article: Feng, D. et al. Kinetically tuned dimensional augmentation as a versatile synthetic route towards robust metal–organic frameworks. Nat. Commun. 5:5723 doi: 10.1038/ncomms6723 (2014). Accession codes: The X-ray crystallographic coordinates for structures reported in this Article have been deposited at the Cambridge Crystallographic Data Centre (CCDC), under deposition number CCDC 975771-975791 and 975820-975828. These data can be obtained free of charge from The Cambridge Crystallographic Data Centre via www.ccdc.cam.ac.uk/data_request/cif .